Evidence for the late formation of hydrous asteroids from young meteoritic carbonates The accretion of small bodies in the Solar System is a fundamental process that was followed by planet formation. Chronological information of meteorites can constrain when asteroids formed. Secondary carbonates show extremely old 53 Mn– 53 Cr radiometric ages, indicating that some hydrous asteroids accreted rapidly. However, previous studies have failed to define accurate Mn/Cr ratios; hence, these old ages could be artefacts. Here we develop a new method for accurate Mn/Cr determination, and report a reliable age of 4,563.4+0.4/−0.5 million years ago for carbonates in carbonaceous chondrites. We find that these carbonates have identical ages, which are younger than those previously estimated. This result suggests the late onset of aqueous activities in the Solar System. The young carbonate age cannot be explained if the parent asteroid accreted within 3 million years after the birth of the Solar System. Thus, we conclude that hydrous asteroids accreted later than differentiated and metamorphosed asteroids. An understanding of the evolution of the asteroid belt can constrain the origin and early history of the Solar System. It is suggested that the accretion time of asteroids determines the degree of metamorphism (and/or melting) they experienced [1] , because a short-lived radionuclide of 26 Al (half-life: 0.73×10 6 years) is the dominant heat source of metamorphism, and hence, the abundance of the heat source is a function of accretion time. Several lines of evidence from the dating of meteorites have shown that the parent bodies of differentiated meteorites accreted earlier than chondrites [2] , [3] . These observations indicate that accretion time is indeed an important controlling factor of asteroidal thermal history, whereas other factors, such as water concentrations in asteroids, could have minor roles. However, the accretion time of hydrous asteroids has been controversial. CM chondrites, which are carbonaceous chondrites named for their type specimen of the Mighei meteorite, experienced aqueous alteration at low temperatures [4] , indicating late accretion. However, the 53 Mn- 53 Cr ages ( 53 Mn decays to 53 Cr with a half-life of 3.7×10 6 years) of the carbonates in CM chondrites revealed by secondary ion mass spectrometry (SIMS) are very old (ref. 5 and references therein), with ages comparable to the oldest solids in the Solar System (that is, calcium-aluminium-rich inclusions (CAIs); 4,568.2 million years ago (Myr ago) [6] ). Although the ages of the secondary minerals in CI chondrites (named for their type specimen of the Ivuna meteorite) may not be as old (4,567 to 4,554 Myr ago [7] , [8] , [9] , [10] , [11] , [12] ), one must conclude that at least some hydrous asteroids, such as the CM chondrite parent body, accreted very rapidly because the accretion time should be constrained by the oldest alteration product. It should be noted, however, that the accuracies of Mn–Cr ages depend on accurate determinations of 55 Mn/ 52 Cr ratios. Accurate 55 Mn/ 52 Cr measurements of meteoritic carbonates require a carbonate standard with a known chemical composition (that is, 55 Mn/ 52 Cr atomic ratio) because the sensitivities of Mn and Cr in SIMS strongly depend on analyte chemical compositions (the so-called 'matrix effect'), and hence, the data obtained for unknown samples should be calibrated using the standard. However, a suitable carbonate standard is not available in natural terrestrial environments, which is why previous studies have used other materials, such as San Carlos olivine, as alternative standards. This use has led to systematic errors on the 55 Mn/ 52 Cr of meteoritic samples and their ages. To overcome this problem, we synthesized a carbonate (calcite: CaCO 3 ) standard doped with Mn and Cr, and we demonstrated that the Mn/Cr relative sensitivity of carbonates is significantly different from that of San Carlos olivine [13] , that is, systematic errors of ~2.2 Myr indeed exist in previous studies for carbonate dating. This result is crucial for a high-resolution chronology of the early Solar System. In the present study, we determined the accurate Mn–Cr ages of carbonates in four CM chondrites using the carbonate standard. We found that the CM carbonates have an identical age of Myr ago, which is younger than previous estimates. The young carbonate age suggests the late onset of aqueous activities in the Solar System. Based on this result, we conclude that the parent asteroid of CM chondrites accreted at ~3.5 Myr after the birth of the Solar System. Initial 53 Mn/ 55 Mn ratios and absolute ages of CM carbonates We performed Mn–Cr isotope measurements of the standard and carbonates in the CM chondrites with different alteration indexes [14] (calcites in Murchison CM 2.5 and Y791198 CM 2.4 and dolomites in ALH83100 CM 2.1 and Sayama CM 2.1) using a NanoSIMS 50. The Mn/Cr relative sensitivity data are presented in Supplementary Figure S1 and Supplementary Table S1 . For all samples, the 53 Cr excesses correlate well with the 55 Mn/ 52 Cr, which indicates the in-situ decay of 53 Mn ( Fig. 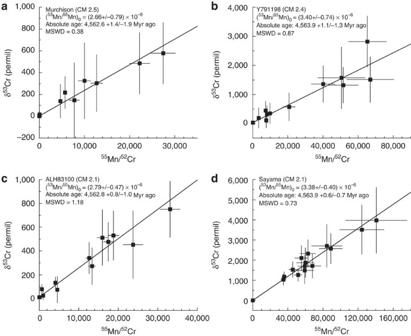Figure 1: Mn–Cr isochron diagrams for carbonates in four CM chondrites. (a) Calcite in the Murchison CM 2.5 chondrite. (b) Calcite in the Y791198 CM 2.4 chondrite. (c) Dolomite in the ALH83100 CM 2.1 chondrite. (d) Dolomite in the Sayama CM 2.1 chondrite. The vertical axis shows53Cr/52Cr described as the permil deviation (δ53Cr) from the value of the synthetic calcite standard. Error bars (±2σ) on both53Cr/52Cr and55Mn/52Cr represent the external reproducibility or the internal precision, whichever is larger. MSWD, mean square weighted deviation. 1 ; Table 1 ). The analyses were performed for several carbonate grains in each meteorite. Hence, it is likely that the carbonates dispersed in each meteorite formed at the same time within the analytical uncertainties. The initial 53 Mn/ 55 Mn ratios, ( 53 Mn/ 55 Mn) 0 , were estimated from the isochron slopes, and the uncertainty in the Mn/Cr relative sensitivity was propagated to the errors on ( 53 Mn/ 55 Mn) 0 . The ( 53 Mn/ 55 Mn) 0 values were found to be (2.59±0.74)×10 −6 , (3.31±0.68)×10 −6 , (2.71±0.40)×10 −6 and (3.28±0.30)×10 −6 for the carbonates in Murchison, Y791198, ALH83100 and Sayama, respectively (errors are 2 σ ). In calculating the absolute ages of carbonates, the LEW 86010 angrite with a known Pb–Pb age [15] and ( 53 Mn/ 55 Mn) 0 (ref. 16 ) was referenced as a time anchor. We assume a homogeneous distribution of 53 Mn in the early Solar System, which is likely to be correct at least among samples from chondrites, the eucrite parent body, Earth and Mars [17] . The initial 53 Mn/ 55 Mn ratios of the carbonates correspond to absolute ages of Myr ago for Murchison, Myr ago for Y791198, Myr ago for ALH83100 and Myr ago for Sayama. Figure 1: Mn–Cr isochron diagrams for carbonates in four CM chondrites. ( a ) Calcite in the Murchison CM 2.5 chondrite. ( b ) Calcite in the Y791198 CM 2.4 chondrite. ( c ) Dolomite in the ALH83100 CM 2.1 chondrite. ( d ) Dolomite in the Sayama CM 2.1 chondrite. The vertical axis shows 53 Cr/ 52 Cr described as the permil deviation ( δ 53 Cr) from the value of the synthetic calcite standard. Error bars (±2 σ ) on both 53 Cr/ 52 Cr and 55 Mn/ 52 Cr represent the external reproducibility or the internal precision, whichever is larger. MSWD, mean square weighted deviation. Full size image Table 1 Mn–Cr isotope data of carbonates in four CM chondrites. Full size table Accuracies of the carbonate ages It should be stressed that we calculated a Cr isotopic ratio by summing all 53 Cr counts, then dividing by the sum of 52 Cr counts over the entire measurement, rather than averaging isotopic ratios (Methods). This is an important difference from earlier studies, that is, an isotope ratio has been traditionally calculated by averaging a number of ratios collected over the course of a measurement, which leads to a positive bias especially in the case of low counting rates [18] . The meteoritic carbonates studied in this study have experienced only low temperatures and it is unlikely that thermally driven volume diffusion has disturbed the Mn–Cr system. Also, other mechanisms of redistribution of the parent and daughter isotopes, such as grain boundary diffusion, can be ruled out because the cathode-luminescence observations of the carbonates show well-preserved zoning of trace elements including Mn. Therefore, we are sure that these ages are indigenous and there are no possibilities of age biases caused by the disturbance of the Mn–Cr system. In summary, we successfully determined the carbonate ages of the CM chondrites, which are free from the potential biases resulting from the matrix-mismatched standard, the calculation of isotopic ratios and/or the disturbance of the Mn–Cr system. It is worth noting that the carbonate ages are younger than those reported previously for the same meteorites. These ages are identical within the errors, irrespective of the degrees of aqueous alteration ( Fig. 2 ). Therefore, we can define a formation age of Myr ago (that is, ~4.8 Myr after CAI formation) for carbonates in CM chondrites using the weighted average. Our data indicate a later accretion of the CM chondrite parent asteroid, and therefore, later onsets of aqueous alteration in the Solar System than previously inferred from the oldest carbonates in the CM chondrites. The problem of the very early formation of carbonates contemporaneous with CAIs is solved using the proper Mn/Cr relative sensitivity. It is also suggested that the carbonates in the CM chondrites precipitated in a relatively short time. This suggestion is contrary to earlier studies suggesting a rough correlation between alteration indexes and carbonate ages of CM chondrites [5] . 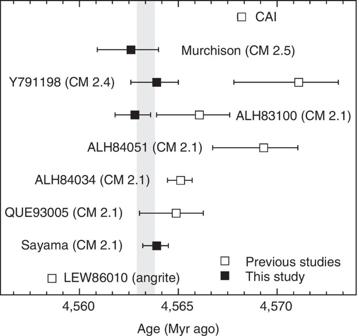Figure 2: Summary and comparison of Mn–Cr ages of carbonates. The filled symbols represent Mn–Cr ages in this study using the calcite standard, and the open symbols represent previously reported data (ref.5and references therein). Also shown are the Pb–Pb age of a type-B CAI from the NWA2364 CV3 chondrite6(named for their type specimen of the Vigarano meteorite) and the Pb–Pb age of the LEW86010 angrite15used as a time anchor. The carbonates in the four CM chondrites analysed here show an identical formation age (; shown by the vertical grey band). Error bars (±2σ) are based on the uncertainties of the Mn/Cr RSF and the isochron slopes (see Methods for details). Figure 2: Summary and comparison of Mn–Cr ages of carbonates. The filled symbols represent Mn–Cr ages in this study using the calcite standard, and the open symbols represent previously reported data (ref. 5 and references therein). Also shown are the Pb–Pb age of a type-B CAI from the NWA2364 CV3 chondrite [6] (named for their type specimen of the Vigarano meteorite) and the Pb–Pb age of the LEW86010 angrite [15] used as a time anchor. The carbonates in the four CM chondrites analysed here show an identical formation age ( ; shown by the vertical grey band). Error bars (±2 σ ) are based on the uncertainties of the Mn/Cr RSF and the isochron slopes (see Methods for details). Full size image Here we consider the accretion time of the CM chondrite parent body. Our new carbonate ages determine the younger side of the accretion time (~4.8 Myr after CAI formation). The older side could be constrained by the 53 Mn- 53 Cr or 26 Al- 26 Mg ages of chondrules. Unfortunately, chondrules in CM chondrites have not been dated yet, and their dating may be complicated by extensive aqueous alteration. Therefore, we rely on the Al–Mg ages of chondrules in CO chondrites (named for their type specimen of the Ornans meteorite), because they are related to CM chondrites in chemical and oxygen isotopic compositions [19] , [20] . Previous studies suggested that the forming events of CO chondrules took place 1.7 to 3.2 Myr after CAI formation [21] , [22] . Thus, the accretion time of the CM chondrite parent body would be 3.2 to 4.8 Myr after the birth of the Solar System. On the basis of the chronological information discussed above, we simulate the thermal history of the CM chondrite parent body and estimate the accretion time. We consider the static water model [20] , [23] here, although the fluid flow model has been investigated in some previous works [24] , [25] , [26] , [27] . The thermal history is modelled using a one-dimensional heat conduction equation in radial form. See Supplementary Methods for details. We assume that an asteroid of 60 km in diameter accreted instantaneously at 3.5 Myr (case A) or 3.0 Myr (case B) after CAI formation, although the results are essentially similar for different asteroid sizes, if the asteroid is larger than 60 km in diameter ( Supplementary Fig. S2 ). The parent body consists of a homogeneous mixture of rock, void space and water ice. The heat source is the decay energy of 26 Al, and the reaction heat of hydration is also included. The parameters and variables used in the model are presented in Supplementary Table S2 and Supplementary Methods . According to the oxygen isotopic compositions [23] and a simulation of chemistry during aqueous alteration [28] , the calcite in Murchison is likely to have precipitated at <25 °C in the earliest stage of aqueous alteration (when less than a few percent of rock reacted with water). The clumped-isotope thermometry also suggests that the calcite in Murchison formed at a low temperature (20–33 °C) [29] . On the other hand, the dolomite in Sayama seems to have formed at a higher temperature (>120 °C), as inferred from the small isotopic fractionation of oxygen between the dolomite and the matrix [30] . In the model set-up described above, the calculated thermal history of case A well reproduces the temperatures of carbonate formation at Myr ago ( Fig. 3a ). In the intermediate region of the asteroid, the peak temperature is less than ~50 °C, and the progress of aqueous alteration is mild. In the inner part, on the other hand, the peak temperature is ~150 °C, and alteration occurs rapidly. While less altered CM chondrites, such as Murchison, could be derived from the outer part of the asteroid, more altered ones, such as Sayama, come from the inner part. In contrast, case B gives a rapid increase in temperature caused by more abundant 26 Al, even if the hydration heat is not considered, and as a consequence, the carbonates are likely to have precipitated at ~4,564.5 Myr ago ( Fig. 3b ). Other heat sources, such as impact heating, inductive heating or decay energies of other radioactive nuclides, if any, would assist the 26 Al heating of the parent body, resulting in a more rapid temperature increase. Therefore, such early accretion as case B is ruled out considering our high-precision Mn–Cr data. Although parameters such as water fraction and the size of the asteroid are not well constrained, it is important to stress that there is no parameter space where carbonates could form at 4.8 Myr after CAI formation, if the parent body accreted within 3.0 Myr after CAI formation, because the timing at which the aqueous alteration began was determined predominantly by the accretion time of the asteroid. 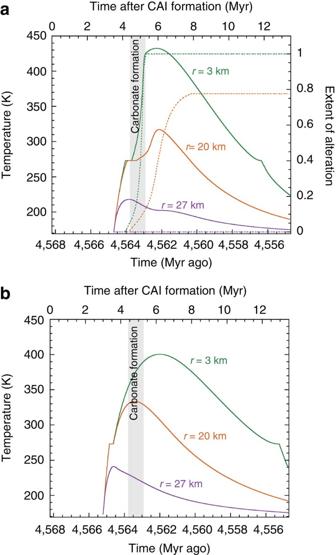Figure 3: Thermal history of CM chondrite parent body without fluid flow. Temperature (solid lines) and the extent of alteration (dotted lines) are given at three depths (r: distance from the centre) in the asteroid with a radius of 30 km. The vertical grey band shows the formation age of carbonates (). (a) Accretion at 3.5 Myr after CAI formation (case A). The extent of alteration is defined by (1−olivineres./olivineini.), where olivineres.and olivineiniare the moles of the residual and initial olivine, respectively. (b) Accretion at 3.0 Myr after CAI formation (case B). Note that the hydration reaction is not included in case B. Figure 3: Thermal history of CM chondrite parent body without fluid flow. Temperature (solid lines) and the extent of alteration (dotted lines) are given at three depths ( r : distance from the centre) in the asteroid with a radius of 30 km. The vertical grey band shows the formation age of carbonates ( ). ( a ) Accretion at 3.5 Myr after CAI formation (case A). The extent of alteration is defined by (1−olivine res. /olivine ini. ), where olivine res. and olivine ini are the moles of the residual and initial olivine, respectively. ( b ) Accretion at 3.0 Myr after CAI formation (case B). Note that the hydration reaction is not included in case B. Full size image An accretion time of >3 Myr after CAI formation is later than the formation of chondrules in the least metamorphosed chondrites (typically ~2 Myr after CAI formation [3] ). On the other hand, the W isotopic compositions of iron meteorites suggest their formation within 1.5 Myr after CAI formation [2] . If the carbonate ages of CI chondrites reported so far also have systematic errors, like those of the CM chondrites, they would become comparable with or younger than the carbonate ages of the CM chondrites [8] , [10] , [11] , [12] . In any case, the early formation of hydrous asteroids suggested by old carbonates in CM chondrites is no longer well founded, and we conclude that hydrous asteroids accreted later than differentiated and metamorphosed asteroids. This conclusion is consistent with the compositional structure of the asteroid belt, which shows that asteroids with spectra indicative of high-temperature silicate minerals are concentrated between 1.8 and 3 AU, whereas dark C-rich types seem to be located farther away from the Sun [31] . NanoSIMS measurement condition We performed the Mn–Cr isotope measurements using a NanoSIMS 50 installed at the Atmosphere and Ocean Research Institute at the University of Tokyo. Both the meteorites and the synthetic calcite standard were embedded in epoxy and polished in the same way. A focused O − primary ion beam of 1 nA was accelerated to 16 keV and irradiated on the surfaces of the samples. Before the measurements, an intense primary beam of ~3 nA was rastered over 20×20 to 50×50 μm 2 on the meteoritic carbonates to remove surface contaminations and to obtain secondary ion images of carbonates to choose measurement spots. Secondary ions were extracted from the sample surfaces by an accelerating voltage of 8 kV, and 43 Ca + , 52 Cr + , 53 Cr + and 55 Mn + ions were detected in a combined peak-jumping/multi-detection mode. The magnet was cycled through two field settings and the waiting times were 2 seconds each. In the first setting, 43 Ca + , 52 Cr + and 55 Mn + were simultaneously detected with three secondary electron multipliers (SEMs). The measurement time was 2 seconds. Subsequently, 53 Cr + was detected with the same SEM as that for 52 Cr + . The measurement time was 5 seconds. The measurements consisted of 150 cycles of the two magnetic field settings. The difference between sensitivities of two SEMs for 52 Cr + and 55 Mn + was corrected when evaluating the Mn/Cr relative sensitivity of carbonates, although this difference was cancelled when we calculated the 55 Mn/ 52 Cr of the meteoritic samples and normalized it to the standard value. The dynamic background of the SEM for 52,53 Cr + was measured by applying a −10 V offset relative to the peak centre on the deflection plates in front of the SEMs. The background ranged from 0.01 to 0.02 cps. Mn/Cr relative sensitivity of carbonates We synthesised a calcite standard doped with Mn and Cr to evaluate the relative sensitivity factor (RSF; defined as ( 55 Mn + / 52 Cr + ) ion /( 55 Mn/ 52 Cr) atomic ) of carbonates. See ref. 13 for details of the production. The synthetic calcite has concentration gradients of Mn and Cr in a single grain. The concentrations decrease from the centre to periphery of a grain due to the fractional crystallization of Mn and Cr. Therefore, we analysed the grains for small regions within 100×100 μm 2 of the grain centre. In these limited areas, the heterogeneities of Mn and Cr are up to 20%. The 55 Mn/ 52 Cr atomic ratios were determined with an electron probe micro analyser (EPMA) around measurement spots with a NanoSIMS. In the EPMA analyses, the Mg, Ca, Cr, Mn and Fe concentrations were determined with a JEOL JXA-8900L. A sample current of 3 nA was accelerated to 15 keV and rastered over ~10×10 μm 2 on the sample surface to avoid damage by electron bombardment. The measurement times of the Mg, Ca, Cr, Mn and Fe concentrations and the background were 10 seconds and 5 seconds, respectively. In the NanoSIMS analyses, we found that the 43 Ca + , 52,53 Cr + and 55 Mn + intensities and the 55 Mn + / 52 Cr + decrease with time for the standard and meteoritic carbonates during a single measurement ( Supplementary Fig. S1 ). This effect is too large to be attributable to the heterogeneities of Mn and Cr in a grain, but rather is due to the charge-up of the calcite. Hence, we used the 'time-dependent RSF' (hereafter described as 'RSF( t )') to calibrate the 55 Mn/ 52 Cr atomic ratios of the meteoritic samples. The RSF( t ) was defined for each measurement cycle (the measurement consisted of 150 cycles of two magnetic field settings). We measured the RSF approximately ten times in each measurement session (the overall measurement consists of three sessions, see Supplementary Fig. S1 and Supplementary Table S1 ), and the average of approximately ten RSF values at a given time (measurement cycle) was used as the RSF( t ) at the time. Then, we calculated the ' 55 Mn + convert. ' of the meteoritic carbonates at a given time as 55 Mn + convert. = 55 Mn + /RSF( t ). Finally, we determined the mean 55 Mn/ 52 Cr atomic ratios of the meteoritic carbonates ( Table 1 ), as 55 Mn/ 52 Cr=Σ( 55 Mn + convert. )/Σ( 52 Cr + ). We did not use the average of the 55 Mn + convert. / 52 Cr + values in the 150 cycles as the mean 55 Mn/ 52 Cr atomic ratio, because the intensity of 52 Cr + was usually quite low, and 55 Mn + convert. / 52 Cr + was often infinite (no 52 Cr + ion was detected in the cycle). The internal errors on 55 Mn/ 52 Cr were calculated as Note that Σ( 55 Mn + ) instead of Σ( 55 Mn + convert. ) was used in calculating the internal error. The uncertainty in the RSF ( σ RSF ) is difficult to estimate. In the three measurement sessions, the average RSF( t ) values are 0.636, 0.675 and 0.690, respectively ( Supplementary Table S1 ). These values vary within 8.1%, although the error in each session is less than 2.4%. This variation seems to be caused by the behaviours of the 55 Mn + / 52 Cr + changes, that is, degrees of charge-up. The degrees of charge-up are likely to be closely related to crater depth produced by primary ion bombardment, which is controlled by the intensity of the primary ion beam in each measurement session. In each measurement session, we found that the change was reproducible, as shown in Supplementary Figure S1 , because we kept the measurement conditions exactly the same including the primary ion beam intensity, which is why the error of the RSF in each session is smaller than the variation among the three sessions. Thus, we are quite sure that the 55 Mn/ 52 Cr of the meteoritic carbonates is properly corrected for the RSF in each measurement session. In this study, we conservatively adopted a σ RSF of 8.1%. We consider that this value can fully describe the uncertainty in the estimated 55 Mn/ 52 Cr ratios, or rather, might be overestimated. This uncertainty was propagated to the final errors on the initial 53 Mn/ 55 Mn ratios, ( 53 Mn/ 55 Mn) 0 , which were calculated as where σ slope is the 95% confident interval of the isochron slope based on and using the York fit program 'Isoplot 3.41' (ref. 32 ). will be defined in the next subsection. Chromium isotope measurements In contrast to the RSF, the Cr isotopic composition is stable for the synthetic calcite standard during a single measurement. The mean values of 53 Cr/ 52 Cr are 0.1103 (1), 0.1102 (3) and 0.1099 (2) in the three measurement sessions, respectively, where the numbers in parentheses represent the uncertainties of the last digits ( Supplementary Table S1 ). We calculated the 53 Cr/ 52 Cr of the meteoritic carbonates as 53 Cr/ 52 Cr=Σ( 53 Cr + )/Σ( 52 Cr + ). We did not use the average of the 53 Cr + / 52 Cr + values in the 150 cycles as the mean 53 Cr/ 52 Cr ratio for the same reason as that for 55 Mn/ 52 Cr. The 53 Cr/ 52 Cr of the meteoritic carbonates is described as the permil deviation ( δ 53 Cr) from the standard value ( Table 1 ). The internal errors on 53 Cr/ 52 Cr ( ) were calculated as How to cite this article: Fujiya, W. et al . Evidence for the late formation of hydrous asteroids from young meteoritic carbonates. Nat. Commun. 3:627 doi: 10.1038/ncomms1635 (2012).